SILAC-based proteomic quantification of chemoattractant-induced cytoskeleton dynamics on a second to minute timescale Cytoskeletal dynamics during cell behaviours ranging from endocytosis and exocytosis to cell division and movement is controlled by a complex network of signalling pathways, the full details of which are as yet unresolved. Here we show that SILAC-based proteomic methods can be used to characterize the rapid chemoattractant-induced dynamic changes in the actin–myosin cytoskeleton and regulatory elements on a proteome-wide scale with a second to minute timescale resolution. This approach provides novel insights in the ensemble kinetics of key cytoskeletal constituents and association of known and novel identified binding proteins. We validate the proteomic data by detailed microscopy-based analysis of in vivo translocation dynamics for key signalling factors. This rapid large-scale proteomic approach may be applied to other situations where highly dynamic changes in complex cellular compartments are expected to play a key role. Directed cell movement is a key mechanism in development and disease and a major question is how the movement of many cells is coordinated and by which mechanisms cells move. Chemotaxis is the best understood mechanism of directed cell movement and improper control and execution plays a major role in a number of diseases including immunological disorders [1] and cancer metastasis [2] . It is a complex process composed of several steps involving signal detection and amplification, cell polarization and cytoskeleton reorganization [3] . The final outcome is actin polymerization at the leading edge driving cellular protrusions and myosin II filament assembly and contractile force generation at the back of the cell [4] . This polarized cytoskeleton organization together with turn-over of the cell-substrate adhesion points lead to chemotactic cell movement. However, there are still many aspects of this complex process that are not fully understood, such as the mechanism of establishing cell polarity in response to external stimuli or coupling the signal transduction to the cytoskeleton reorganization. Studies in genetically tractable model organisms such as Dictyostelium show that dynamic spatiotemporal changes in the actin–myosin cytoskeleton are regulated by multiple parallel evolutionarily highly conserved signalling pathways of considerable complexity [5] , [6] , [7] . In many cases, chemoattractants are detected via G protein coupled seven transmembrane receptors, which activate the members of Ras and Rho families of small GTPases [8] , [9] , [10] . Ras signalling is directly activated by the Gβγ complex and is a master regulator of several downstream signal transduction pathways such as the PI3 kinase and TorC signalling pathways [11] , [12] . Members of the Rho family of small GTPases, working as components of the signalling pathways downstream of Ras, are specialized regulators of the actin–myosin cytoskeleton dynamics [13] , [14] . These proteins act as molecular switches cycling between active GTP-bound and inactive GDP-bound states, which are controlled by a large family of specific regulatory factors [15] . Guanine-nucleotide exchange factors promote activation of small GTPases while GTPase-activating proteins mediate their transition to the inactive state [16] . Only activated small GTPases can interact with downstream effectors and regulate their function. It has been observed that fast moving cells such as Dictyostelium amoebae and human neutrophils exhibit a rapid biphasic actin polymerization [17] , [18] , [19] and a slower myosin II assembly/translocation response [20] , [21] after stimulation with a suitable chemoattractant. In Dictyostelium, the first rapid phase of actin polymerization is independent of PI3K/PTEN signalling and occurs uniformly throughout the whole cortex [17] . It is followed by a fast depolymerization phase after which the second slower phase of actin polymerization occurs. This second slower response, which is confined to regions of pseudopodia extension, is known to require PI3K/PTEN signalling [17] . It would appear that this highly synchronous response to chemoattractant stimulation is a good system to dissect the temporal dynamics of the actin–myosin cytoskeleton. Here we describe an unbiased proteomic approach to quantify changes in the composition of the cortical cytoskeleton and associated proteins during the chemotactic response with a second timescale resolution. We establish the stable isotope labelling by amino acids in cell culture (SILAC) procedure for use in Dictyostelium and utilize it to perform a large-scale quantitative analysis of protein translocation dynamics. We validate our results by in vivo imaging of selected regulatory factors tagged with fluorescent proteins. These methods allow us to obtain novel interesting insights in the role of major signalling components and the temporal scale on which they act. SILAC-based quantitative analysis of protein translocation The standard procedure for measuring the dynamic changes in the cytoskeleton during chemotactic response involves isolation of crude detergent insoluble cell fractions at different times after chemoattractant stimulation, followed by analysis of these fractions for specific proteins [22] . To perform this analysis on a proteome-wide scale, we have adapted the SILAC technique [23] for Dictyostelium to obtain labelled and unlabelled cell populations. One population is stimulated with cAMP and rapidly lysed at different times, while the lysates from the other unstimulated population are added in equal proportions to each time point to serve as an internal reference of protein abundance during mass spectrometry analysis. We first established whether the SILAC methodology can be used to label the proteome of Dictyostelium cells. We analysed the labelling efficiency of cells grown in defined media supplemented with K8 L -lysine and R6 L -arginine after five rounds of cell divisions. We found that both amino acids were efficiently incorporated into the proteome with the average labelling efficiency of 93% ( Fig. 1 ). We did not detect any significant arginine to proline transition in this organism. Dictyostelium is a very robust organism adapted to live in the soil and thrives in a wide range of temperatures. We performed the chemoattractant stimulation experiments at 12 °C, which slows down the responses and allows reproducible sample collection of the early time points. Under these conditions, the fast response peaks at 10 s followed by a depolymerization phase lasting until 60 s, while the second response shows a very broad peak lasting from ~100 s to ~240 s ( Fig. 2a ). We prepared cell lysates before stimulation and at 1, 4 and 10 s after stimulation to catch the rising phase of the first response. The 20 and 60 s time points represent depolymerization phase while 120 and 180 s time points represent the second phase of actin polymerization. Crude cytoskeletal preparations, which contained around 10 percent of the total protein from the lysates, were fractionated using SDS–PAGE followed by tryptic in-gel digest [24] and peptide extraction. Proteomic analyses were performed using LTQ-Velos Orbitrap tandem mass spectrometer and the data processing and quantification were done by MaxQuant [25] software ( Fig. 2c ). Protein light/heavy (L/H) ratios were quantified in each time point based on a minimum of two different peptide ratios. Out of around 2,500 identified proteins over 1,800 proteins passed the detection threshold, with ratios quantified in at least four out of eight time points. Based on the Gene Ontology annotations only about 200 of those proteins were known cytoskeletal components, while the remaining proteins belonged to other cellular compartments or were of unknown function and localization. It is no surprise that we find many components of different organelles since the detergent insoluble fractions contain, besides the filamentous actin–myosin cytoskeleton, also other cellular structures resistant to lysis such as nuclei and mitochondria. Many highly and medium abundant proteins not related to the cytoskeleton, such as aquaporins or nucleopore components, showed only small temporal changes in abundance, rarely exceeding 20% of the pre-stimulation values. We obtained a data set of 472 proteins after filtering the proteins that showed a significant similarity (Pearson’s correlation >0.2) in the temporal kinetics of the two replica experiments and a temporal variation in relative abundance greater than 40% to ensure reliability of the profiles. Ninety-nine proteins had a cytoskeletal GO component annotation ( Fig. 2d ). Figure 2 shows the individual temporal profiles of these cytoskeletal proteins in the heat-map format. 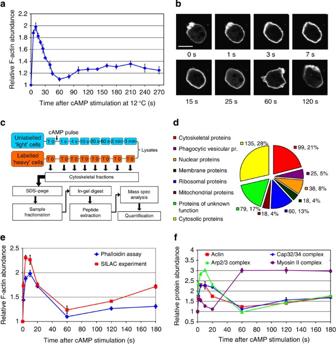Figure 2: Cytoskeletal dynamics during chemotactic response and SILAC experimental approach. (a) Graph of actin polymerization dynamics after cAMP stimulation measured at 12 °C using the phalloidin assay. Graph represents a mean of 15 measurements and error bars represent standard error of the mean (s.e.m.). (b) Confocal images of a cell expressing LifeAct-RFP at different time points after cAMP stimulation. The 1-s, 3-s, 7-s time points correspond to the 1st phase of actin polymerization, 15 and 25 s to the actin depolymerization phase, 60 and 120 s to the 2nd polymerization phase. Scale bar, 10 μm. (c) Workflow chart of the SILAC experiment. Unlabelled cells are stimulated with cAMP at 12 °C and lysed at various time points after stimulation. Lysates are mixed in equal proportions with SILAC cell lysates from unstimulated cells. Crude cytoskeletal fractions are processed by separation on SDS–PAGE and gels fractionation followed by in-gel tryptic digest. Peptides are analysed using tandem mass spectrometry. The mass spec data are processed and quantified by Mascot and MaxQuant. (d) Distribution of Gene Ontology (GO) term annotations in the filtered data set of detected proteins showing reproducible temporal enrichment profiles. Values indicate number of proteins in each GO component annotation group and percentage of the total number of proteins in the filtered data set. (e) Comparison of the actin polymerization dynamics profiles measured in the phalloidin assay (blue) and the SILAC experiments (red). Blue graph represents the mean of 15 measurements and red graph represents mean of two biological replicates of the SILAC experiment, error bars represent s.e.m. (f) Protein incorporation dynamics of the major structural components of the cytoskeleton. Graphs show temporal enrichment profiles for actin (red—same as ine), Arp2/3 (green), Cap32/34 (blue) and myosin II (purple) protein complexes. All the graphs except for actin, represent means of the enrichment values for all the subunits of each protein complex from two biological replicates of the SILAC experiment, error bars represent s.e.m. Of interest are also 79 unknown proteins showing a reproducible enrichment profile after cAMP stimulation that we have identified here. Eight of those proteins were validated as novel cytoskeletal associated/interacting factors by GFP-tagging and in vivo imaging. 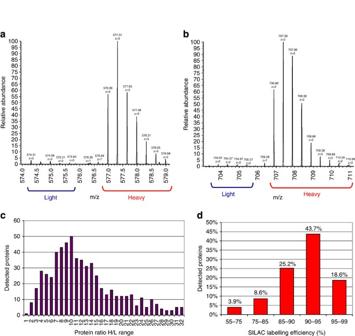The function of these unknown proteins is currently being analysed through targeted gene disruption experiments. Figure 1: SILAC labelling efficiency inD. discoideum. (a) Mass spectrum (MS) of a peptide containing a single lysine residue (ALHLFGPTLGYFGEAK) with heavy/light (H/L) ratio value of 29.7. (b) MS of a peptide containing a single arginine residue (AAITNDFIGSEIR) with H/L ratio value of 51.9. Blue brackets indicate isotopic distribution peaks belonging to the ‘light’ forms and red brackets to the ‘heavy’ forms. (c) Protein H/L ratios distribution of 616 detected proteins. H/L ratio 4 indicates a 80% labelling efficiency, H/L ratio 9 indicates 90% labelling efficiency and H/L ratio 19 indicates 95% labelling efficiency etc. (d) Labelling efficiency distribution of all the detected proteins. The analysed sample came from a cell population grown in a defined medium containing K8 L-lysine and R6 L-arginine for five rounds of cell doubling. Figure 1: SILAC labelling efficiency in D. discoideum . ( a ) Mass spectrum (MS) of a peptide containing a single lysine residue (ALHLFGPTLGYFGEA K ) with heavy/light (H/L) ratio value of 29.7. ( b ) MS of a peptide containing a single arginine residue (AAITNDFIGSEI R ) with H/L ratio value of 51.9. Blue brackets indicate isotopic distribution peaks belonging to the ‘light’ forms and red brackets to the ‘heavy’ forms. ( c ) Protein H/L ratios distribution of 616 detected proteins. H/L ratio 4 indicates a 80% labelling efficiency, H/L ratio 9 indicates 90% labelling efficiency and H/L ratio 19 indicates 95% labelling efficiency etc. ( d ) Labelling efficiency distribution of all the detected proteins. The analysed sample came from a cell population grown in a defined medium containing K8 L-lysine and R6 L-arginine for five rounds of cell doubling. Full size image Figure 2: Cytoskeletal dynamics during chemotactic response and SILAC experimental approach. ( a ) Graph of actin polymerization dynamics after cAMP stimulation measured at 12 °C using the phalloidin assay. Graph represents a mean of 15 measurements and error bars represent standard error of the mean (s.e.m.). ( b ) Confocal images of a cell expressing LifeAct-RFP at different time points after cAMP stimulation. The 1-s, 3-s, 7-s time points correspond to the 1st phase of actin polymerization, 15 and 25 s to the actin depolymerization phase, 60 and 120 s to the 2nd polymerization phase. Scale bar, 10 μm. ( c ) Workflow chart of the SILAC experiment. Unlabelled cells are stimulated with cAMP at 12 °C and lysed at various time points after stimulation. Lysates are mixed in equal proportions with SILAC cell lysates from unstimulated cells. Crude cytoskeletal fractions are processed by separation on SDS–PAGE and gels fractionation followed by in-gel tryptic digest. Peptides are analysed using tandem mass spectrometry. The mass spec data are processed and quantified by Mascot and MaxQuant. ( d ) Distribution of Gene Ontology (GO) term annotations in the filtered data set of detected proteins showing reproducible temporal enrichment profiles. Values indicate number of proteins in each GO component annotation group and percentage of the total number of proteins in the filtered data set. ( e ) Comparison of the actin polymerization dynamics profiles measured in the phalloidin assay (blue) and the SILAC experiments (red). Blue graph represents the mean of 15 measurements and red graph represents mean of two biological replicates of the SILAC experiment, error bars represent s.e.m. ( f ) Protein incorporation dynamics of the major structural components of the cytoskeleton. Graphs show temporal enrichment profiles for actin (red—same as in e ), Arp2/3 (green), Cap32/34 (blue) and myosin II (purple) protein complexes. All the graphs except for actin, represent means of the enrichment values for all the subunits of each protein complex from two biological replicates of the SILAC experiment, error bars represent s.e.m. Full size image The actin polymerization dynamics detected in the SILAC experiments closely matches the results from other standard biochemical assay used to measure this process ( Fig. 2e ). The major constituents of the cytoskeleton, actin and myosin II, were the most abundant proteins in the cytoskeletal preparations. The dynamic patterns of these and other structural proteins, such as the actin nucleator Arp2/3 and capping protein Cap32/34 complexes, showed excellent agreement with previously reported biochemical data [22] , [26] . Arp2/3 and Cap32/34 complexes follow the biphasic actin dynamics during the chemotactic response. The temporal dynamics of myosin II, which is known to have a different pattern of translocation with a long lasting peak during the second phase of actin polymerization [20] , is also well reproduced in the proteomic analysis ( Fig. 2f ). In all cases, the different subunits of these protein complexes showed very similar dynamics. Overall, these findings strongly validate the experimental approach taken here. There are several important general conclusions about cytoskeletal dynamics that can be drawn from the SILAC data set. First, it is very clear that even though two actin nucleators of the Formin family were detected and showed a reproducible biphasic association patterns, the Arp2/3 complex was far more abundant and showed a much stronger enrichment in both phases after cAMP stimulation ( Supplementary Data 1 , 2 , 3 and 4 ). This strongly indicates that the Arp2/3 complex is the main nucleator of actin filaments in both phases of cAMP-dependent actin polymerization. Following the same logic, we can conclude that the Cap32/34 complex, which is the only detected actin capping protein, is the main factor responsible for capping the fast growing ends of actin filaments in chemotaxing cells and that it binds as soon as filaments start to form. In fact, a similar argument can be applied to nearly all the cytoskeletal factors identified in the proteomic experiments, where only few members of each class or family were detected. In order to determine whether this partial detection of only some family members was due to differences in protein abundance or in differences in binding to the cytoskeleton, we performed a quantitative proteomic analysis of the total cell lysates from the ‘heavy’ cell population mixed with an equal amount of protein from the detergent insoluble fraction of the ‘light’ population. We used finer fractionation to improve proteome coverage in this sample, and we indeed managed to detect almost one thousand additional proteins in this experiment. For some families, we detected additional members as in the case of the Rab subfamily of small GTPases and the syntaxin proteins of the t-SNARE family, both involved in vesicle trafficking. We also detected some actin binding proteins such as gelsolin-related proteins ( Supplementary Data 5 ). As expected there were also some protein families such as RacGEF’s, for which fewer members were detected in this experiment, due to the lower enrichment of these factors in the total lysate and the higher complexity of this sample. The experiment clearly showed the different levels of enrichment or depletion of proteins in the insoluble fraction, indicating distinct binding characteristics for each protein. A major factor in determining protein detection during mass spec analysis of complex samples is their abundance. Given that proteins within a certain class or family often show high levels of redundancy in function, a selective detection of only some members may suggest that these are likely to be the major actors performing specific functions in for instance the capping or bundling of actin filaments. A typical example is provided by the family of Elmo proteins, known interactors of the Dock family of RacGEF’s [27] . ElmoE, which has been described as a key component of the signalling pathway regulating actin cytoskeleton [28] , is the only Elmo protein detected in our SILAC experiments. It shows a strong response to cAMP stimulation ( Fig. 3b ) and therefore is likely a key member of this family in the regulation of cytoskeletal dynamics in chemotaxing cells. In Dictyostelium, there are 45 proteins containing RacGEF domains encoded in the genome [14] . We reproducibly detected 16 in our experiments and all exhibited a cAMP-dependent translocation dynamics. Similarly 7 out of 46 RacGAP’s were detected and showed dynamic response to cAMP stimulation ( Fig. 3b ). These cytoskeletal regulatory factors exhibit cAMP driven association with the cytoskeletal cortex and based on the detection levels from our unbiased proteomic studies likely represent key members of these protein classes in the control of cytoskeletal dynamics. 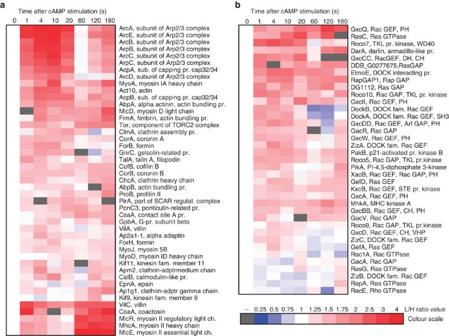Figure 3: Heat-map representation of the temporal incorporation profiles for the cytoskeletal proteins detected in the SILAC experiments. (a) Structural and effector proteins of the cytoskeleton. (b) Factors involved in the signalling pathways controlling cytoskeletal dynamics. Heat-maps show proteins that were detected in two biological replica experiments showing positive correlation (R>0.2) between the temporal dynamics detected in each experiment. Columns represent time points after the cAMP stimulation. Red colour indicates increase of protein abundance and blue colour indicates depletion from the cytoskeletal fraction based on the L/H protein ratios normalized to the pre-stimulation value (heat-map colour scale illustrates quantitation). White represents a pre-stimulation level (t0=1) and grey indicates lack of data (protein not detected in any experiment at this time point). On the right side of the heat-maps are given names of the proteins with a brief annotation. It describes protein function (for example, actin bundling protein), protein class (for example, RacGEF or TKL protein kinase), name of the protein complex for subunits (for example, Arp2/3 or myosin II), and names of the major domains of regulatory components. Protein profiles were clustered with Cluster3 software and heat-maps were generated with Java TreeView software. Figure 3: Heat-map representation of the temporal incorporation profiles for the cytoskeletal proteins detected in the SILAC experiments. ( a ) Structural and effector proteins of the cytoskeleton. ( b ) Factors involved in the signalling pathways controlling cytoskeletal dynamics. Heat-maps show proteins that were detected in two biological replica experiments showing positive correlation (R>0.2) between the temporal dynamics detected in each experiment. Columns represent time points after the cAMP stimulation. Red colour indicates increase of protein abundance and blue colour indicates depletion from the cytoskeletal fraction based on the L/H protein ratios normalized to the pre-stimulation value (heat-map colour scale illustrates quantitation). White represents a pre-stimulation level ( t 0 =1) and grey indicates lack of data (protein not detected in any experiment at this time point). On the right side of the heat-maps are given names of the proteins with a brief annotation. It describes protein function (for example, actin bundling protein), protein class (for example, RacGEF or TKL protein kinase), name of the protein complex for subunits (for example, Arp2/3 or myosin II), and names of the major domains of regulatory components. Protein profiles were clustered with Cluster3 software and heat-maps were generated with Java TreeView software. Full size image DockA and DockB show the fastest response of all RacGEF’s We detected three major temporal patterns of protein enrichment in the cytoskeletal fraction in our SILAC experiments. The most common pattern, shared by a diverse range of cytoskeletal effectors and regulators, is an actin-like biphasic profile. The other two patterns are formed by proteins that show enrichment mainly during either the first or the second phase of actin polymerization ( Fig. 3 ). These patterns are less frequent but very informative since they may suggest a specific role of the relevant proteins in one of the two phases. Signalling factors that showed incorporation mainly during the first phase of actin polymerization include DockA, DockB, ZizC, GxcD, GefA, Roco7 and Roco9. DockA and DockB are Dock180-related proteins from the CZH family of unconventional RacGEF’s, which have been implicated in several cytoskeleton-related processes, including cell migration and phagocytosis [29] , [30] , [31] . DockA has been reported to be involved in the regulation of actin cytoskeleton during cell migration in Dictyostelium [32] . ZizC is another member of the same CZH family of RacGEF’s [30] but it has not yet been characterized. GxcD is a multi-domain protein containing a RacGEF domain [14] as well as two actin binding domains (ABD’s): calponin homology and villin headpiece domains [33] . GefA (Aimless) is a RasGEF responsible for activation of RasC downstream of cAMP receptor and it is involved in the regulation of chemotaxis and cAMP relay response in Dictyostelium [34] , [35] . Roco7 and Roco9 belong to a large and evolutionarily conserved family of multi-domain proteins characterized by having a unique combination of a Ras-like GTPase domain called Roc, a unique COR (C-terminal of Roc) domain and a serine–threonine protein kinase domain, Roco9 contains an additional RacGAP domain. Roco proteins are involved in a diverse range of cellular functions including cell divisions, cell polarity, chemotaxis and development [36] , [37] , [38] . Both Roco7 and Roco9 are expressed mostly during the aggregation stage in Dictyostelium [36] . The identification of this set of regulatory factors forms one of the most interesting outcomes of the current SILAC experiments. These proteins are most likely involved in triggering the rapid process of global cytoskeletal reorganization following cAMP stimulation. DockA and DockB show the highest association at the earliest time point of the first phase of the response ( Fig. 4a,d ), which suggests that these two RacGEF’s are among the earliest regulators responding to the chemoattractant stimulation and therefore are likely to be placed close to the receptor in the signalling pathway. 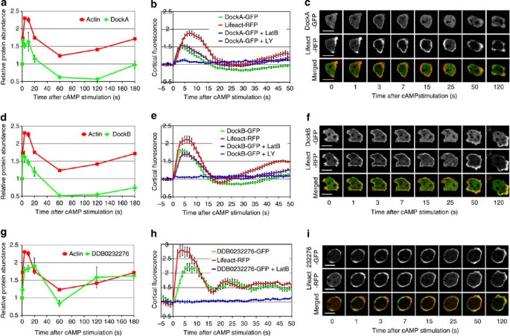Figure 4: Comparison of SILAC-based protein dynamics with thein vivodynamics of GFP-tagged proteins. Results for three proteins of interest: DockA (a–c); DockB (d–f) and a novel protein DDB0232276 (g–i). (a,d,g) Protein translocation dynamics measured in the SILAC experiments. Incorporation profiles of the analysed proteins (green) compared with F-actin dynamics (red). Graphs represent means from two biological replicates and error bars represent s.e.m. (b,e,h) Protein translocation measured by confocal imaging of cells co-expressing GFP-tagged proteins together with Lifeact-RFP. Graphs represent quantification of cortical fluorescence intensity relative to the cytosolic fluorescence intensity and normalized to the pre-stimulation time point. Both GFP signal (green) and RFP signal (red) were measured simultaneously during response to cAMP stimulation. Blue lines indicate GFP signal quantification from cells stimulated with cAMP at the presence of 15 μM Latrunculin B. Purple lines indicate GFP signal quantification from cells stimulated in the presence of 80 μM LY294002. Data shown are means and standard errors (s.e.) for a minimum of 10 cells measured in at least two different experimental days. (c,f,i) Micrographs of confocal imaging of stimulated cells from selected time points representing peaks of different phases of actin polymerization dynamics. GFP channel is shown in the top row, RFP channel in the middle and merged channel in the bottom row of each panel. Scale bars, 10 μm. See alsoSupplementary Movies 1,2and3. Figure 4: Comparison of SILAC-based protein dynamics with the in vivo dynamics of GFP-tagged proteins. Results for three proteins of interest: DockA ( a – c ); DockB ( d – f ) and a novel protein DDB0232276 ( g – i ). ( a , d , g ) Protein translocation dynamics measured in the SILAC experiments. Incorporation profiles of the analysed proteins (green) compared with F-actin dynamics (red). Graphs represent means from two biological replicates and error bars represent s.e.m. ( b , e , h ) Protein translocation measured by confocal imaging of cells co-expressing GFP-tagged proteins together with Lifeact-RFP. Graphs represent quantification of cortical fluorescence intensity relative to the cytosolic fluorescence intensity and normalized to the pre-stimulation time point. Both GFP signal (green) and RFP signal (red) were measured simultaneously during response to cAMP stimulation. Blue lines indicate GFP signal quantification from cells stimulated with cAMP at the presence of 15 μM Latrunculin B. Purple lines indicate GFP signal quantification from cells stimulated in the presence of 80 μM LY294002. Data shown are means and standard errors (s.e.) for a minimum of 10 cells measured in at least two different experimental days. ( c , f , i ) Micrographs of confocal imaging of stimulated cells from selected time points representing peaks of different phases of actin polymerization dynamics. GFP channel is shown in the top row, RFP channel in the middle and merged channel in the bottom row of each panel. Scale bars, 10 μm. See also Supplementary Movies 1 , 2 and 3 . Full size image Validation of the SILAC results by in vivo protein imaging In order to validate the incorporation patterns detected in the SILAC experiments 30 cytoskeletal proteins were tagged with GFP and visualized in vivo using confocal and total internal reflection fluorescence (TIRF) microscopy. All of them exhibited cortical localization and various levels of cAMP-dependent translocation to the cortex. Since the proteomic experiments and the imaging analysis were performed at different temperatures, the timing of protein translocation was somewhat different and could only be compared in reference with actin dynamics. The GFP-tagged proteins were therefore co-expressed with RFP-tagged LifeAct probe staining F-actin structures [39] allowing simultaneous measurement of actin polymerization dynamics. The protein translocation dynamics observed in vivo was generally in excellent agreement with the proteomic data. Confocal and TIRF imaging of DockA and DockB confirmed the very early onset of the translocation peak of those proteins after cAMP stimulation. Both RacGEF’s show a significantly faster rate of translocation to the cortex than the rate of actin polymerization, which is most clearly visible for DockA ( Fig. 4a–f , Supplementary Movies 1 , 2 ). A different translocation pattern is exhibited by one of the novel cytoskeletal factors detected in the SILAC experiment and validated by in vivo imaging—protein DDB0232276. In both proteomic and microscopy measurements, this protein shows a slower kinetics compared with the first phase of actin polymerization and has a broad peak of enrichment lasting until the middle of the actin depolymerization phase ( Fig. 4g–i , Supplementary Movie 3 ). This uncharacterized protein contains an ADF/cofilin-like domain, suggesting a possible role in F-actin depolymerization, which would be supported by its translocation kinetics. Further examples of microscopy-based validation of the SILAC dynamics are shown for three known regulators of the cytoskeletal dynamics—PakB [40] , [41] , KxcB [14] and RapGAP1 (refs 42 , 43 ) ( Fig. 5 ). In order to verify the F-actin-dependent nature of the protein translocation, we measured the translocation response to cAMP stimulation in the presence of the actin polymerization inhibitor—15 μM Latrunculin B. The translocation of all analysed proteins was blocked by this inhibitor, which confirmed that their association with the cytoskeleton is driven by binding to cortical F-actin structures ( Figs 4 , 5 ). In addition, we checked whether incorporation of DockA and DockB is regulated by PI3K signalling, since it has been reported that DockD, the other member of this family of RacGEF’s, shows a phosphatidylinositide (3,4,5) phosphate (PIP3)-dependent translocation [32] . Confocal imaging studies demonstrate that translocation of DockA and DockB is not suppressed by the PI3K inhibitor—80 μM LY294002, indicating a PIP3 independent type of incorporation to the cortex ( Fig. 4b,e ). 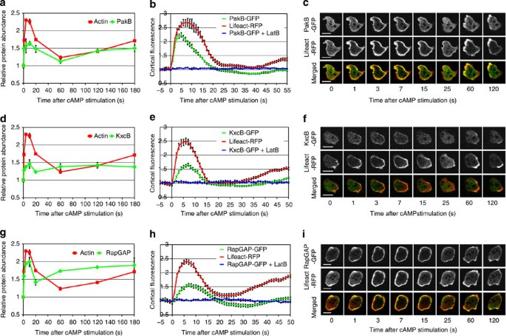Figure 5: Comparison of SILAC-based protein dynamics with thein vivodynamics of GFP-tagged proteins. Results for three proteins of interest: PakB (a–c); KxcB (d–f) and RapGAP1 (g–i). (a,d,g) Protein translocation dynamics measured in the SILAC experiments. Incorporation profiles of the analysed proteins (green) compared with F-actin dynamics (red). Graphs represent means from two biological replicates and error bars represent s.e.m. (b,e,h) Protein translocation measured by confocal imaging of cells co-expressing GFP-tagged proteins together with Lifeact-RFP. Graphs represent quantification of cortical fluorescence intensity relative to the cytosolic fluorescence intensity and normalized to the pre-stimulation time point. Both GFP signal (green) and RFP signal (red) were measured simultaneously during response to cAMP stimulation. Blue lines indicate GFP signal quantification from cells stimulated with cAMP at the presence of 15 μM LatrunculinB. Data shown are means and s.e. for a minimum of 10 cells measured in at least two different experimental days. (c,f,i) Micrographs of confocal imaging of cAMP-stimulated cells at selected time points representing peaks of the different phases of actin polymerization dynamics. The GFP channel is shown in the top row, the RFP channel in the middle and the merged channel in the bottom row of each panel. Scale bars, 10 μm. Figure 5: Comparison of SILAC-based protein dynamics with the in vivo dynamics of GFP-tagged proteins. Results for three proteins of interest: PakB ( a – c ); KxcB ( d – f ) and RapGAP1 ( g – i ). ( a , d , g ) Protein translocation dynamics measured in the SILAC experiments. Incorporation profiles of the analysed proteins (green) compared with F-actin dynamics (red). Graphs represent means from two biological replicates and error bars represent s.e.m. ( b , e , h ) Protein translocation measured by confocal imaging of cells co-expressing GFP-tagged proteins together with Lifeact-RFP. Graphs represent quantification of cortical fluorescence intensity relative to the cytosolic fluorescence intensity and normalized to the pre-stimulation time point. Both GFP signal (green) and RFP signal (red) were measured simultaneously during response to cAMP stimulation. Blue lines indicate GFP signal quantification from cells stimulated with cAMP at the presence of 15 μM LatrunculinB. Data shown are means and s.e. for a minimum of 10 cells measured in at least two different experimental days. ( c , f , i ) Micrographs of confocal imaging of cAMP-stimulated cells at selected time points representing peaks of the different phases of actin polymerization dynamics. The GFP channel is shown in the top row, the RFP channel in the middle and the merged channel in the bottom row of each panel. Scale bars, 10 μm. Full size image DockA and DockB co-localize to the same cortical structures The proteomic analysis revealed that DockA and DockB share virtually identical and very unique translocation profiles, which suggests that they might form a protein complex or bind to the same structures. Protein co-localization studies from dual-channel TIRF microscopy confirmed that these two closely related RacGEF’s show the same kinetics of incorporation to the cortex after cAMP stimulation as well as a very strong co-localization determined by Pearson’s correlation coefficient ( R =0.8) ( Figs 6a,b and 7a and Supplementary Movie 4 ). However, the observed slower dissociation of DockB from the cortex compared with DockA does not support the formation of a constitutive stable protein complex. Dock proteins are known to activate Rac GTPases [44] that act through SCAR complex [45] to result in activation of the Arp2/3 complex [46] and actin polymerization. To probe the role of DockA/B in this pathway, we performed co-localization studies of DockA with SCAR. These experiments revealed a strong co-localization (Pearson’s correlation R =0.6) and similar timing of translocation of these two proteins ( Figs 6c,d and 7b and Supplementary Movie 5 ). 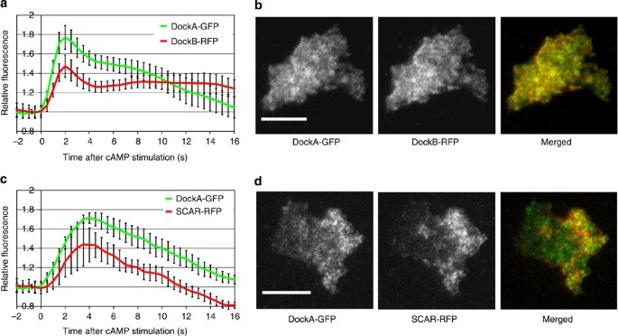Figure 6: Co-localization analysis from dual-channel TIRF microscopy. DockA-GFP was co-expressed with DockB-RFP (a,b) and SCAR-RFP (c,d). Both GFP and RFP signals were simultaneously imaged using TIRF microscope with an image splitter at two frames per second (fps). (a,c) Quantification of cAMP-induced translocation dynamics. Graphs represent average fluorescence intensity from the cell area normalized to the pre-stimulation time point. Data shown are means and s.e. for a minimum of 10 cells measured in at least two different experimental days. (b,d) Micrographs from the TIRF imaging showing cells at the peak of the 1st phase of actin polymerization. GFP channel is shown on the left, RFP channel in the middle and merged channel on the right. Scale bars, 10 μm. See alsoFig. 7andSupplementary Movies 4,5. Figure 6: Co-localization analysis from dual-channel TIRF microscopy. DockA-GFP was co-expressed with DockB-RFP ( a , b ) and SCAR-RFP ( c , d ). Both GFP and RFP signals were simultaneously imaged using TIRF microscope with an image splitter at two frames per second (fps). ( a , c ) Quantification of cAMP-induced translocation dynamics. Graphs represent average fluorescence intensity from the cell area normalized to the pre-stimulation time point. Data shown are means and s.e. for a minimum of 10 cells measured in at least two different experimental days. ( b , d ) Micrographs from the TIRF imaging showing cells at the peak of the 1st phase of actin polymerization. GFP channel is shown on the left, RFP channel in the middle and merged channel on the right. Scale bars, 10 μm. See also Fig. 7 and Supplementary Movies 4 , 5 . 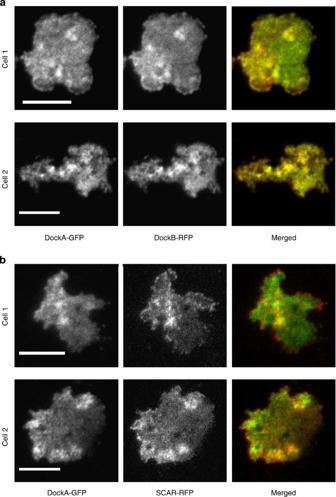Figure 7: Co-localization data from dual-channel TIRF microscopy. DockA-GFP was co-expressed with DockB-RFP (a) and with SCAR-RFP (b). Both fluorescence signals were simultaneously imaged using TIRF microscope with an image splitter at 2 fps. TIRF micrographs from both co-localization studies show two different cells at the peak of the 1st phase of actin polymerization. The GFP channel is shown on the left, the RFP channel in the middle and the merged channel on the right of each panel. Scale bars, 10 μm. Full size image Figure 7: Co-localization data from dual-channel TIRF microscopy. DockA-GFP was co-expressed with DockB-RFP ( a ) and with SCAR-RFP ( b ). Both fluorescence signals were simultaneously imaged using TIRF microscope with an image splitter at 2 fps. TIRF micrographs from both co-localization studies show two different cells at the peak of the 1st phase of actin polymerization. The GFP channel is shown on the left, the RFP channel in the middle and the merged channel on the right of each panel. Scale bars, 10 μm. Full size image DockA and DockB are key activators of actin polymerization To directly verify whether DockA and DockB are important regulators of the first phase of chemotactic response as indicated by our SILAC experiments, we generated and analysed single and double knockout strains. Analysis of cAMP-induced actin polymerization dynamics revealed that both docA − and docB − single knockouts showed decreased levels of F-actin during the first phase. The double docA − /docB − mutant showed a synergistic phenotype with the lowest levels of actin polymerization during the first phase ( Fig. 8a ). These results confirmed that both of these RacGEF’s are involved in activation of the rapid actin polymerization response and indicated a redundancy in their function during this process. Differences in F-actin levels between the single mutants in the second phase response may indicate separate functions during this phase of the chemotactic response. The Dock knockout strains showed decreased velocity during random motility of vegetative cells, while cells overexpressing either DockA or DockB showed strongly elevated levels of movement velocity ( Fig. 8b ). These phenotypes of the dock mutants indicate that both DockA and DockB proteins play a role in the regulation of cell motility, which is in agreement with the in vivo imaging studies showing their localization at the leading edge of the pseudopodia ( Fig. 4c,f : 120 s) and with the previously reported data for DockA [32] . Even though the proteomic analysis did not show enrichment of Dock proteins in the second phase ( Fig. 4a,d ) the imaging data show a clear translocation during this phase. The discrepancy between the SILAC and imaging results most likely indicates a change of binding affinity or a change of interaction during the response. 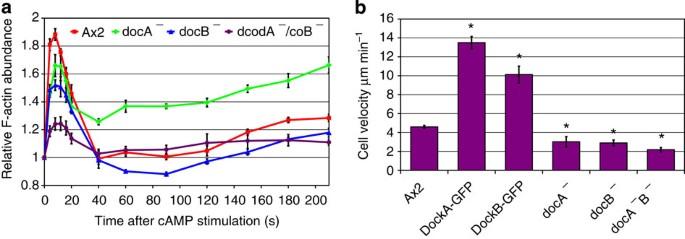Figure 8: Phenotypes of deletion and overexpression of Dock proteins. (a) cAMP-dependent actin polymerization response measured in wild-type (Ax2) cells (red),docAKO cells (green),docBKO cells (blue) anddocA/docBdouble KO cells (purple). Graph shows quantification of actin bands in the cytoskeletal fractions separated by SDS–PAGE and stained with fluorescent protein dye—Krypton. Plots represent means and s.e. of four separate experiments normalized to the pre-stimulation time point. (b) Velocity data of wild-type strain (Ax2), strains overexpressing Dock proteins and knockout mutants. Vegetative cells expressing LifeAct-RFP were imaged with confocal microscope during random walk for 20 min; their velocity was quantified using Quimp software. Bars represent average velocities and s.e. from at least 15 cells. The overexpressors showed statistically significant (t-test) increased velocity (Ax2/DockA (P=5.4e−14), Ax2/DockB, (P=3.6e−7)) and the knockouts were significantly slower (Ax2/docA−(P=1e−2), Ax2/docB−(P=1e−4), Ax2/docA−docB−(P=4.9e−7)) compared with wild-type Ax2cells. Figure 8: Phenotypes of deletion and overexpression of Dock proteins. ( a ) cAMP-dependent actin polymerization response measured in wild-type (Ax 2 ) cells (red), docA KO cells (green), docB KO cells (blue) and docA/docB double KO cells (purple). Graph shows quantification of actin bands in the cytoskeletal fractions separated by SDS–PAGE and stained with fluorescent protein dye—Krypton. Plots represent means and s.e. of four separate experiments normalized to the pre-stimulation time point. ( b ) Velocity data of wild-type strain (Ax 2 ), strains overexpressing Dock proteins and knockout mutants. Vegetative cells expressing LifeAct-RFP were imaged with confocal microscope during random walk for 20 min; their velocity was quantified using Quimp software. Bars represent average velocities and s.e. from at least 15 cells. The overexpressors showed statistically significant ( t -test) increased velocity (Ax 2 /DockA ( P =5.4e −14 ), Ax 2 /DockB, ( P =3.6e −7 )) and the knockouts were significantly slower (Ax 2 /docA − ( P =1e −2 ), Ax 2 /docB − ( P =1e −4 ), Ax 2 /docA − docB − ( P =4.9e −7 )) compared with wild-type Ax 2 cells. Full size image Protein cross-linking identifies new interactions Our standard SILAC experimental procedure detects relatively high affinity protein–protein interactions that are stable throughout the sample preparation period and will not detect more transient interactions, which may also be relevant. In order to overcome this problem, we have tested several protein cross-linkers in pilot experiments. We obtained the largest increase in number of detected proteins after formaldehyde fixation during cell lysis followed by thermal reversal of formaldehyde cross-linking. The latter procedure was used to repeat the standard experiment. This showed that the majority of abundant cytoskeletal proteins detected in the standard experiment were also detected and showed similar kinetics after formaldehyde cross-linking ( Fig. 9 ). Some of the large multi-subunit proteins such as myosin II showed similar dynamics but somewhat lower amplitudes of enrichment, most likely caused by incomplete reversal of the cross-linking preventing their successful separation on SDS–PAGE. The most interesting part of this complementary data set is a group of about 70 cytoskeleton-related proteins that were not detected in the standard experiments ( Fig. 10 ). This group includes some actin binding proteins such as Severin A and Formin A, but also known membrane associated proteins such as PTEN [47] and phospholipase C [48] . About half of the proteins in this group exhibit enrichment during the second phase of actin polymerization. The most straightforward interpretation of this result is that these proteins play a specific role during the second phase of the response as for instance in the case of RacC. This Rac GTPase has been previously shown to be an important regulator of actin polymerization and PI3K activation specifically during the second phase of the chemotactic response [49] . There were five members of class I myosin family, which were detected only in the cross-linked SILAC, while there were a further three class I myosins that were detected in both types of preparation. These actin-based molecular motors mediate interactions between the cytoskeleton and the plasma membrane. A few of them detected exclusively in the cross-linked experiment were shown to bind to PIP3 (ref. 50 ). The fact that most of class I myosins could be detected only in the cross-linked SILAC suggests that their affinity to the cytoskeleton is relatively weak. There were few types of G protein alpha subunits detected only in this experiment indicates that they also interact with the cytoskeleton with low affinity. Another interesting result is the detection of SCAR protein, NapA and AbiA subunits of the SCAR complex, which is a major activator of the actin nucleator Arp2/3 complex [46] , [51] , [52] , only in the cross-linked SILAC. Another component of the SCAR complex, PirA was detected in both types of the SILAC experiments ( Figs 9 , 10 ). These observations imply that from all the subunits of the SCAR complex only the regulatory subunit PirA forms stable interactions with the cytoskeleton. DockD, another member of Dock family in Dictyostelium implicated in the control of actin dynamics [32] , was also detected only in the cross-linked SILAC experiment. 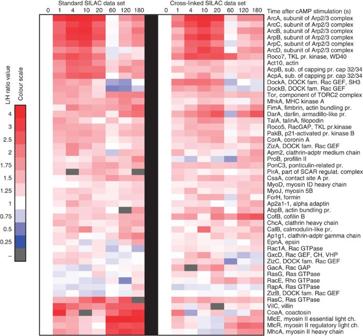Figure 9: Comparison of the temporal incorporation profiles detected in the standard and cross-linked SILAC experiments. Temporal enrichment profiles from the standard SILAC experiments (left) are paired with the profiles detected in the cross-linked SILAC experiment (right). Heat-maps represent cytoskeletal proteins that showed positive correlation (R>0.2) between the incorporation profiles detected in those two types of SILAC experiments. Columns represent time points after the cAMP stimulation. Red colour indicates increase of protein abundance and blue colour indicates depletion from the cytoskeletal fraction based on the L/H protein ratios normalized to the pre-stimulation value (heat-map colour scale illustrates quantitation). White represents a pre-stimulation level (t0=1) and grey indicates lack of data. Protein profiles were clustered with Cluster3 software and heat-maps were generated with Java TreeView software. Figure 9: Comparison of the temporal incorporation profiles detected in the standard and cross-linked SILAC experiments. Temporal enrichment profiles from the standard SILAC experiments (left) are paired with the profiles detected in the cross-linked SILAC experiment (right). Heat-maps represent cytoskeletal proteins that showed positive correlation (R>0.2) between the incorporation profiles detected in those two types of SILAC experiments. Columns represent time points after the cAMP stimulation. Red colour indicates increase of protein abundance and blue colour indicates depletion from the cytoskeletal fraction based on the L/H protein ratios normalized to the pre-stimulation value (heat-map colour scale illustrates quantitation). White represents a pre-stimulation level ( t 0 =1) and grey indicates lack of data. Protein profiles were clustered with Cluster3 software and heat-maps were generated with Java TreeView software. 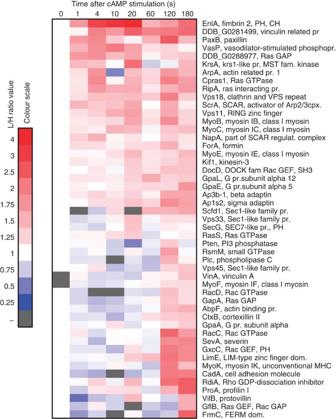Figure 10: Temporal incorporation profiles for the proteins detected only in the cross-linked SILAC experiment. Heat-map represents cytoskeleton-related proteins that were detected only after formaldehyde cross-linking of the analysed samples and were not detected in the standard SILAC experiments. Heat-map description as before. Full size image Figure 10: Temporal incorporation profiles for the proteins detected only in the cross-linked SILAC experiment. Heat-map represents cytoskeleton-related proteins that were detected only after formaldehyde cross-linking of the analysed samples and were not detected in the standard SILAC experiments. Heat-map description as before. Full size image The described results show that the SILAC-based proteomics method is capable of unbiased measurement of changes in protein association dynamics for hundreds to thousands of proteins in a single experiment on a second to minute timescale. This feature provides a great advantage over other biochemical (for example, western blot) and imaging methods used for this type of studies, which can only analyse few proteins at a time and are often dependent on a biased approach of protein tagging and overexpression. The protein translocation dynamics observed in vivo by fluorescence microscopy analyses was generally in excellent agreement with the proteomic data; however, for some proteins, the results were not strongly correlated. This is most likely due to the overexpression-related phenotypes observed in some strains used for microscopy studies. The proteomic method used here detects proteins that are stably incorporated into the structures of the actin–myosin cytoskeleton such as actin, myosin II and Arp2/3 as well as interacting proteins such as capping protein and actin bundling proteins. The detected protein–protein interactions can by highly dynamic but must have a relatively high affinity to persist during sample preparation. It is likely that the affinity of some proteins is high enough to show an observable translocation in vivo , but too low to be detected in the proteomic analysis under native conditions. This is the likely reason that some of the known interactors like class I myosins were only detected in the cross-linked experiment, where some protein–protein interactions are rapidly stabilized during and after lysis. Overall, these experiments have given important insights into the relative dynamics of major cytoskeletal proteins during chemoattractant-driven changes in the actin–myosin cytoskeleton in a single experiment. We have identified a number of regulators of small GTPases showing association with the cytoskeleton specifically during the first or the second phase of the chemotactic response. Two RacGEF’s, DockA and DockB were validated as key activators of the first phase of actin polymerization by mutational analysis and in vivo microscopy-based localization studies. The SILAC-based proteomic method described here allowed discovery of unknown proteins whose kinetics suggested that they are involved in the analysed process. We have now several of these novel cytoskeletal proteins under further investigation, which will undoubtedly result in obtaining further insight in the control and dynamics of the cytoskeleton. This method is easily extendable to other cell types and chemoattractants and can also be readily generalized for the investigation of other interesting fast biological responses that can be synchronized by a defined trigger, such as phagocytosis, endocytosis and cell division. Materials Complete HL-5 and defined SIH (-arginine; -lysine) growth media and unlabelled L -arginine and L -lysine were from Formedium. Labelled K8 L -lysine and R6 L -arginine were from Cambridge Isotope Laboratories. Complete EDTA-free protease inhibitor cocktail was from Roche. Turbo DNase was from Ambion. Novex NuPAGE 4–12% gradient bis-tris gels with MOPS SDS running buffer and Novex colloidal blue staining kit were from Invitrogen. Trypsin Gold was from Promega. LavaPep peptide quantification kit was from Gel Company. ZipTip C-18 peptide purification microcolumns and high fidelity KOD hot start DNA polymerase were from Merck Millipore. Restriction enzymes, T4 DNA ligase and Antarctic phosphatase were from New England Biolabs. Plasmid miniprep kit and PCR clean-up kit were from Qiagen. Krypton fluorescent protein stain and Nunc Lab-Tek chambered cover glass plates for cell imaging were from Thermo Scientific. All the other reagents were obtained from Sigma-Aldrich. Cell growth and stimulation in the SILAC experiments Dictyostelium Ax 2 cells were grown in suspension until the populations went through six cell doublings. One population was grown in a ‘light’ SIH medium and the other in a ‘heavy’ medium with L -lysine and L -arginine substituted with K8 L -lysine and R6 L -arginine. Cells were harvested at the density of 5 × 10 6 cells per ml, washed twice with development buffer (5 mM KH 2 PO 4 5 mM Na 2 HPO 4 , 2 mM MgSO 4 , 0.4 mM CaCl 2 , pH 6.2) and resuspended in DB at the density of 1 × 10 7 cells per ml. Cells were developed on a rotary shaker for 5 h by pulsing with 30 nM final concentration of cAMP at 6-min intervals. Developed cells were washed once with DB without calcium (DB−Ca ++ : 5 mM KH 2 PO 4 5 mM Na 2 HPO 4 , 2 mM MgSO 4 , pH 6.2) containing 1 mM EGTA, then once with DB-Ca ++ and resuspended at the final density of 2 × 10 7 cells per ml in DB-Ca ++ cooled to 12 °C containing 3 mM caffeine to inhibit endogenous cAMP oscillations [53] . After 20 min incubation at 12 °C, the ‘light’ cells were transferred to a 50-ml falcon tube and placed in a 12 °C water bath on a magnetic stirrer rotating at about 300 r.p.m. in a 4 °C cold room. Cells were stimulated with cAMP at a final concentration of 5 × 10 −4 M. Five-hundred microliter samples were transferred into 2-ml tubes containing 500 μl of ice-cold 2 × lysis buffer (1 × LB: 20 mM HEPES pH 7.4, 2 mM EGTA pH 8, 2 mM MgCl 2 , 0.2% Triton X-100, 1 × protease inhibitors cocktail) shaking on a horizontal mixer (IKA, Vibrax VXR). Samples were taken before and 1, 4, 10, 20, 60, 120 and 180 s after the cAMP stimulation. One ml of the ‘heavy’ cell lysate, prepared by mixing 5 ml of unstimulated ‘heavy’ cells with 5 ml of ice-cold 2 × LB and vortexing for 20 s, was transferred into each ‘light’ sample. The resulting mixed lysates were centrifuged for 2 min at 20,000 g at 2 °C. Pellets were resuspended in 1 ml of ice-cold wash buffer (100 mM HEPES pH 7.4, 2 mM MgCl 2 , 1 × protease inhibitors cocktail) and transferred into 1.5 ml protein LoBind (Eppendorf) tubes and centrifuged again as above. The resulting pellets were frozen until further processing. Cross-linked SILAC protocol All the cell growth and development conditions were the same as described above. In the cross-linked SILAC experiment, the stimulation of ‘light’ cells was repeated four times. A total of 125 μl samples were collected for each time point in each stimulation and lysed with equal volume of ice-cold 2 × fixing lysis buffer (1 × : 20 mM HEPES pH 7.4, 2 mM EGTA pH 8, 2 mM MgCl 2 , 0.2% Triton X-100, 1% formaldehyde) and kept on ice for 30 min. The cross-linking reaction was quenched by adding Tris-HCl pH 8 to the final concentration of 350 mM. The lysates of corresponding time points from all 4 stimulation experiments were pooled. The ‘heavy’ cell lysate was prepared as described above but with Fixing LB and was incubated on ice for 30 min and quenched as above before mixing with the pooled ‘light’ cell lysates. After centrifugation, the pellets were washed twice with 1 ml of wash buffer. For the reversal of formaldehyde, cross-linking samples were boiled with sample buffer (100 mM Tris pH 8, 4% SDS, 25 mM DTT, 5 mM EDTA, 4.5% glycerol) at 99 °C for 40 min. Determination of cytoskeletal enrichment factor All the cell growth and development conditions were the same as described above. After development 1 × 10 7 cells from the ‘heavy’ population was centrifuged and lysed in 20 μl of 1.5 × Turbo DNase buffer containing 1% Triton X-100. 3 × 10 7 cells from the ‘light’ population was centrifuged and resuspended in 0.5 ml of DB-Ca ++ and lysed by mixing with 0.5 ml of ice-cold 2 × LB. Insoluble fraction was centrifuged and washed once with 1 ml of wash buffer. Final pellet was resuspended in 20 μl of 1.5 × Turbo DNase buffer. Two units of Turbo DNase and 100 ng of RNase A were added to both samples, which were then incubated at 37 °C for 30 min. Samples were solubilized by adding 10 μl of 4 × SB without DTT and protein concentration was determined using DC Protein Assay Kit (Bio-Rad). Hundred microgram of proteins from both samples were mixed and processed following the standard procedure described below with increased fractionation into 24 instead of 12 fractions. Sample preparation and mass spectrometry analysis The pellets (~7 μl) were resuspended in 12 μl of 1.5 × Turbo DNase buffer supplemented with 1 × protease inhibitors cocktail containing 2 units of Turbo DNase and 100 ng of RNase A and were incubated at 37 °C for 30 min. Samples were then mixed with 7 μl of 4 × SB and boiled at 96 °C for 6 min. Proteins were alkylated with 3 μl of fresh 1 M iodoacetamide by incubating at room temperature in the dark for 30 min. Ten microliters of 4 × urea buffer (1 × UB: 100 mM Tris pH 8, 1% SDS, 2 M urea, 4.5% glycerol, 0.02% bromophenol blue) was added to obtain the final sample volume of ~40 μl. Proteins were separated on 10 well, 1.5-mm thick, NuPAGE 4–12% bis-tris gradient gels and stained with Novex colloidal blue staining kit in a sterile 14 cm tissue culture dish. Sample lanes were cut into 12 fractions and each gel fraction was further cut into 1 × 1 mm cubes and transferred into individual 1.5 ml Protein LoBind tube. Gel pieces were washed with 500 μl of 40 mM (NH 4 ) 2 CO 3 and mixed on a horizontal mixer at 1,500 r.p.m. for 15 min. A quantity of 500 μl of CH 3 CN was added and samples were incubated at 45 °C for 2 h with periodic mixing. The supernatant was discarded and 250 μl of CH 3 CN was added to dehydrate the gel pieces for 10 min. The supernatant was discarded and gel pieces were dried in a vacuum centrifuge (Thermo Scientific, Savant SPD131DDA) for 10 min. Dried gel pieces were covered with 50 μl of 40 mM (NH 4 ) 2 CO 3 containing 10 μg ml −1 of Trypsin Gold and incubated at room temperature for 30 min to rehydrate. Between 30 and 100 μl of 40 mM (NH 4 ) 2 CO 3 was used to cover the gel pieces completely and samples were incubated at 37 °C overnight [24] . Peptides were extracted with equal volumes (80–150 μl) of 50% CH 3 CN/0.1% trifluoroacetic acid by incubating at 45 °C for 3 h with periodic mixing on a horizontal mixer at 1,500 r.p.m. Supernatants were transferred to fresh Protein LoBind tubes and 400 μl of 50% CH 3 CN/0.1% TFA was added to the gel pieces followed by incubation at 45 °C for 2 h with periodic mixing. Combined supernatants were evaporated in a vacuum centrifuge at 45 °C until fully dry. Dried peptides were resuspended in 15 μl of 0.1% TFA and purified using ZipTip C-18 peptide purification microcolumns following the recommended procedure. Final peptide concentration was measured using LavaPep peptide quantification kit and 1 μg of peptides was used for mass spectrometry analysis. Liquid chromatography–mass spectrometry analysis were performed using Ultimate 3000 nano-HPLC system (Dionex) coupled through nanoelectrospray ionization emitter (New Objective) with LTQ-Velos Orbitrap tandem mass spectrometer (Thermo Scientific). Peptides were separated on a 150 mm × 75 μm Acclaim PepMap C-18 reverse phase column (Dionex) over a 100 min run with a flow rate of 300 nl min −1 of organic gradient. After leaving the column peptides were ionized with nanoelectrospray at 1.2 kV. Proteomic data analysis Raw MS and MS/MS data were processed and quantified using MaxQuant [25] version 1.0.13.13 software and Mascot Daemon version 2.3.2 (Matrix Science) was used to search peptides in the Dictyostelium protein database. Data were analysed with the following settings: two missed cleavages allowed, enzyme used was trypsin, 0.5 kDa mass tolerance for fragment ions, maximum 0.05 PEP value for peptide identification. One fixed modification: Carbamidomethylation (C); and few variable modifications were selected: Oxidation (M); acetylation (N-term); phosphorylation (S,T,Y). Protein ratios were determined based on a minimum of two peptide ratios using razor and unique peptides. Detected proteins were annotated in Excel with Gene Ontology annotations and detailed protein information obtained from the DictyBase. Only proteins that had ratios quantified in at least four time points per experiment were filtered for further analysis. For each protein the L/H ratios were first normalized to their average value over the time series in each experiment and then two replica experiments were merged by averaging ratios for each time point and s.e. were calculated. The final protein ratio series were normalized to the pre-stimulation time point whenever available, and s.e. were recalculated. Time series from the cross-linked SILAC were normalized to the pre-stimulation values whenever available. Pearson’s correlation coefficient between the temporal profiles from different SILAC experiment was calculated and used to filter the proteins based on the reproducibility of the results. In order to estimate the measurement background noise we analysed profiles of over 100 proteins that were expected to be detected but not responding to the chemoattractant stimulation, such as subunits of nucleopore, histone variants and porins. These relatively abundant proteins showed average changes around 15% of the pre-stimulation values with standard deviations (s.d.) around 8–12% at different time points. These fluctuations were considered a good representation of the measurement background noise and only changes at least two s.d. higher than this level, which corresponds to around 35% of the pre-stimulation values, were considered reliable. The final normalized and filtered time series were analysed using Cluster3 software [54] by centroid linkage clustering using City-Block distance as a similarity metric. Heat-maps were generated using the Java TreeView software [55] . Phalloidin actin polymerization assay To measure the actin polymerization in response to cAMP stimulation, we used a modified version of the method previously described [56] . Cells grown in HL-5 medium were harvested at the density of 4 × 10 6 cells per ml and were developed and stimulated as described above. Stimulation was performed at 12 °C water bath in the cold room. A total of 200 μl samples collected before and in various time points after the cAMP stimulation were lysed with equal volumes of ice-cold 2 × fixing LB containing 500 nM Phalloidin-TRITC. Lysates were mixed on a horizontal mixer at 700 r.p.m. in the dark at RT for 2 h. Samples were centrifuged at 20,000 g at 10 °C for 10 min. Phalloidin-TRITC was extracted from the pellets with 500 μl of methanol for 1 h at RT on a horizontal mixer. Samples were centrifuged at 20,000 g at RT for 2 min and two replicas of 200 μl for each time point were transferred to a 96-well flat transparent microtiter plate. Rhodamine fluorescence was measured using microtiter plate fluorometer (Anthos2001, Anthos Labtech) with 540 nm excitation filter and 575 nm emission filter. Construction of GFP expression vectors We have modified the Dictyostelium discoideum extra-chromosomal amino- and carboxy-terminal GFP expression vectors pDM317 and pDM323 (ref. 57 ) by introducing new restriction sites and extending the linker region followed by introduction of a LifeAct-RFP expression cassette under the control of the actin15 promoter. The linker region was changed by adding AgeI restriction site between the two existing sites for BglII and SpeI in the multiple cloning sites. At the same time, the linker fragment between the insert and the C-term GFP tag on pDM323 was extended from four amino acids (ThrSerSerGly) to eight amino acids (ThrSerAlaGlyAlaSerSerGly). The five amino acid linker (SerGlyLeuArgSer) on pDM317 was not modified. These modifications were made by inserting short fragments of dsDNA formed from oligos with cohesive ends compatible with BglII and SpeI restriction sites present on the vectors. The mRFPmars-LifeAct (RFP-LifeAct) expression cassette was created by inserting dsDNA fragment encoding 20 aa long LifeAct probe into the BglII and SpeI sites on pDM318 with N-term mRFPmars tag [57] . The whole expression cassette with act15 promotor, RFP-LifeAct construct and act8 terminator was amplified by PCR using high fidelity KOD polymerase with primers introducing NgoMIV restriction sites at the ends of the cassette. The NgoMIV digested, purified PCR product was cloned into the NgoMIV restriction site on the modified pDM317 and pDM323 vectors. Molecular cloning procedures Genes selected for cloning were amplified from genomic DNA by PCR using KOD polymerase and primers, which introduced restriction sites at the ends of the PCR products (see Supplementary Table 1 ). Each forward primer contained restriction site for BglII or one of the enzymes generating compatible cohesive ends: BamHI or BclI. Several genes, which had internal sites for all the above restriction enzymes, were cloned using AgeI site. Reverse primers were carrying restriction sites for SpeI or XbaI or NheI. All the restriction sites on the primers were flanked with five base fragments to allow efficient digest of the PCR products. Primers were designed to have the annealing temperature of 54 °C. All the genes were amplified using standard PCR conditions with 24 cycles, annealing temperature of 50 °C, annealing time of 15 s, extension temperature of 68 °C and extension time of 40 s per kb. For a few genes the number of cycles was increased up to 28. Reactions were performed in 50 μl with 30 ng of genomic DNA and 0.5 unit of KOD polymerase in Eppendorf Mastercycler ep Gradient S. PCR products were purified and digested simultaneously with two restriction enzymes appropriate for each construct’s design after restriction digest samples were purified again and the DNA concentration was measured with NanoDrop ND 1000 spectrophotometer (Thermo Scientific). These final samples were ligated into previously generated vectors, which were digested with SpeI and BglII or AgeI and dephosphorylated with Antarctic phosphatase. A quantity of 30 ng of plasmid DNA was mixed with approximately two molar excess of insert DNA in 5 μl samples. Ligations were performed using 0.5 unit of T4 DNA ligase at 16 °C overnight and the whole sample volumes were used for transformation of chemo-competent DH5 Escherichia coli cells. Generated clones were screened by colony PCR with primers amplifying the whole insert with GFP-tag and the final constructs were verified by restriction analyses. Construction of docA and docB knockout constructs DocA (DDB_G0291974) 1361–4205, bp sequence was amplified and cloned into pCR-Blunt II-TOPO (Invitrogen). To make the disruption construct the hygromycin cassette was cut from pHygAK-REMI/TOPO by XbaI and SacI and was cloned blunt end into the BaeI site in docA sequence. DocB (DDB_G0270404) 5245–6755, bp sequence was amplified and cloned into pCR-Blunt II-TOPO. To make the disruption construct the Cre-BSR cassette was cut from pLPBLP by SmaI [58] and cloned blunt end into the BstBI site in docB . The disruption constructs were amplified by PCR using the same primers (see Supplementary Table 1 ) and transfected into Ax 2 cells followed by selection with hygromycin (50 μg ml −1 ) and blasticidin (7.5 μg ml −1 ), respectively. Transformants were selected and targeted integration was checked by PCR and southern blot. Dictyostelium transfection AX 2 cells were grown in a shaking culture in HL-5 medium up to 4 × 10 6 cells per ml. Cells were harvested by centrifugation at 600 g for 2 min, washed two times with ice-cold H-50 buffer (20 mM HEPES pH 7, 50 mM KCl, 10 mM NaCl, 1 mM MgSO 4 , 5 mM NaHCO 3 , 1 mM NaH 2 PO 4 , pH 7) and resuspended in H-50 buffer at the density of 5 × 10 7 cells per ml. A quantity of 100 μl of this cell suspension was mixed with 1 μg of plasmid DNA and transferred to an ice-cold 0.1 cm electroporation cuvette. Cells were electroporated with two 0.65 kV pulses at 25 μF capacitance with 5-s interval [59] . Cuvettes were incubated on ice for 5 min and the cells were transferred to HL-5 medium with ampicillin and streptomycin. To select stable transformants, G418 was added 6–12 h after transfection to a final concentration of 30 μg ml −1 . In vivo fluorescence microscopy Cells from each strain were developed as described before. After development, cells were washed once with DB-Ca ++ containing 1 mM EGTA then with DB and resuspended in DB with 3 mM caffeine. Hundred microliters of these cell suspensions was transferred to separate chambers of 8-chambered cover glass and mixed with additional 250 μl of DB with 3 mM caffeine. Cells were kept in the dark for 10 min and were then used for imaging with confocal and TIRF microscopy. During each imaging session, cells were stimulated by adding 50 μl of 1 mM cAMP to the chamber. Confocal microscopy Dual-excitation confocal microscopy was performed using a Leica SP2 confocal laser scanning microscope with a 100 × 1.3 NA oil immersion objective at 512 × 512 pixel resolution. GFP was exited at 488 nm and emitted light was collected between 495–535 nm. mRFPmars was exited at 543 nm and emitted light collected at 580–640 nm. Both channels were detected simultaneously at 1 fps with 800 Hz scanner speed. Cortical fluorescence dynamics and cell motility were quantified from confocal images by Quimp plugin [60] to the Fiji software [61] . TIRF microscopy Dual-channel TIRF microscopy was performed using Nicon Eclipse T i TIRF microscope with 100 × 1.45 NA objective equipped with an OptoSplit II image splitter (Cairn Optics). GFP was exited at 488 and emitted light detected at 500–530 nm. mRFPmars was exited at 594 nm and fluorescence was detected at 600–680 nm. Both channels were detected simultaneously by a Photometrics CascadeII EMCCD camera at 1,024 × 1,024 pixels resolution with exposure times between 100 and 300 ms at 2 fps. Co-localization between two channels was quantified using Coloc2 plugin to the Fiji software [61] . How to cite this article : Sobczyk, G. J. et al . SILAC-based proteomic quantification of chemoattractant-induced cytoskeleton dynamics on a second to minute timescale. Nat. Commun. 5:3319 doi: 10.1038/ncomms4319 (2014). Accession codes: Raw proteomic data have been deposited in the PRIDE Archive under accession code PXD000738 .